Whole-genome sequencing of bladder cancers reveals somaticCDKN1Amutations and clinicopathological associations with mutation burden Bladder cancers are a leading cause of death from malignancy. Molecular markers might predict disease progression and behaviour more accurately than the available prognostic factors. Here we use whole-genome sequencing to identify somatic mutations and chromosomal changes in 14 bladder cancers of different grades and stages. As well as detecting the known bladder cancer driver mutations, we report the identification of recurrent protein-inactivating mutations in CDKN1A and FAT1. The former are not mutually exclusive with TP53 mutations or MDM2 amplification, showing that CDKN1A dysfunction is not simply an alternative mechanism for p53 pathway inactivation. We find strong positive associations between higher tumour stage/grade and greater clonal diversity, the number of somatic mutations and the burden of copy number changes. In principle, the identification of sub-clones with greater diversity and/or mutation burden within early-stage or low-grade tumours could identify lesions with a high risk of invasive progression. Bladder cancer is the seventh most common cancer in the developed world, with tobacco smoking a major cause ( http://www.wcrf.org/cancer_statistics/developed_countries_cancer_statistics.php ). Management of non-muscle-invasive and/or low-risk disease (pTa, papillary, or flat carcinoma in situ ) focuses on prevention of progression and identification of patients likely to develop high-risk tumours (pT1G3, high grade, invading lamina propria) in order to offer them early, aggressive intervention, including radical cystectomy [1] . However, there is a likelihood of overtreating some pTa or pT1 tumours that would never have progressed to the more life-threatening muscle-invasive disease (pT2+, invading muscularis propria). Two different genetic T1G3 sub-types have been reported, one derived from pTa disease with FGFR3 and HRAS overexpression and/or mutations, and the other from flat carcinoma in situ with TP53 , RB1 and PTEN mutations and/or loss [2] . Whole-exome sequencing of bladder tumours has recently identified mutations of chromatin-remodelling genes, such as KDM6A and MLL3 (ref. 3 ), and of STAG2, which encodes a protein involved in sister chromatid cohesion [4] , [5] , [6] . Moreover, four mutation signatures, principally comprising different combinations of C:G>T:A and G:C>C:G substitutions, have been detected in some bladder cancers, although their origins remain unclear [7] . Whole-genome sequence data at sufficiently high depth for comprehensive variant calling have not previously been reported for bladder cancers. Here we perform whole-genome sequencing of bladder cancers of various stages and grades to search for driver mutations, chromosome-scale somatic changes, mutation signatures and clonal structures. We report the identification of mutations in the p53 effector CDKN1A (p21 WAF1/CIP1 ) and the protocadherin FAT1, describe the genomic landscape of the set of cancers, and detect associations between tumour stage and measures of mutation burden. 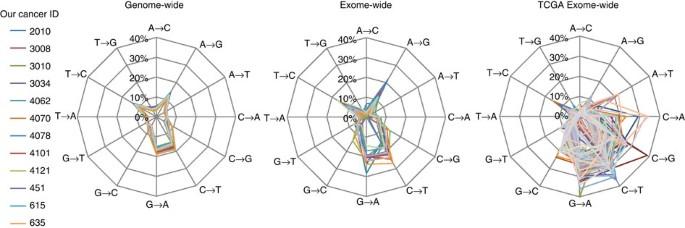Figure 1: Somatic SNV spectrum genome-wide. The proportions of somatic SNVs of each type are shown for each of our cancers (whole genome or exome) in comparison with the TCGA bladder cancer data (exomes). Overview of the bladder cancer genome Our discovery set for whole-genome sequencing comprised 14 bladder cancers ( Table 1 ), which were sequenced at a median depth of ~80 × , alongside paired constitutional DNA from peripheral blood. Making use of the Stampy and Platypus programs for mapping, aligning and calling variants, the number of somatic base substitution mutations (single nucleotide variants (SNVs)) called with high confidence ranged from 27,490 to 121,016 per cancer (median=88,215). Of these, a median of 219 changes (range 82–585) were potentially functional (non-synonymous, splice site, stop-gain or stop-loss) substitutions within protein-coding regions. The mean non-synonymous:synonymous mutation ratio was 1.76. 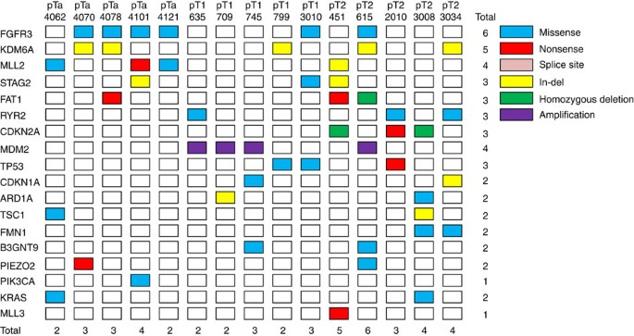Figure 2: Summary of known and putative somatic-driver mutations after filtering in each cancer. MDM2amplification is included in the figure for comparison withTP53andCDKN1A.The established driver mutationsPIK3CAandMLL3are included despite being present in only one tumour to allow comparison with the presence of other mutations. Note that only mutations passing our filtering criteria are shown here, and that other potentially pathogenic mutations of lesser predicted functional effects may exist in these cancers. Other mutation summary statistics are shown in Table 2 and Supplementary Table 1 . Table 1 Demographic and clinicopathological features of the patients and their bladder cancers. Full size table Table 2 Summary genome profiles of the cancers. Full size table The genome-wide SNV spectrum ( Fig. 1 ) showed no single predominant mutation type, with C:G>T:A changes being most common, followed by T:A>C:G and C:G>G:C. This mutation spectrum was broadly similar across all 14 tumours ( Fig. 1 ; Supplementary Fig. 1 ) and was significantly different from all the four recently described bladder cancer mutation signatures (1b, 2, 5 and 13) [7] . However, our mutation spectrum was similar to signature 1b, related to spontaneous demethylation of methyl cytosine, across most substitutions apart from G:C>A:T and C:G>G:C. The signature profiles of the somatic mutations in our samples differed subtly at the exomic and genome-wide levels ( Fig. 1 ). C:G>T:A changes, for example, were more common in the exome than whole genome (41 versus 33%, respectively), perhaps reflecting the greater G:C content in the former. Figure 1: Somatic SNV spectrum genome-wide. The proportions of somatic SNVs of each type are shown for each of our cancers (whole genome or exome) in comparison with the TCGA bladder cancer data (exomes). Full size image The number of high-confidence somatic insertion–deletion (indel) mutations of a few base pairs (bp) ranged from 5,118 to 26,407 per tumour (median=21,704). There was a strong correlation between the numbers of SNVs and indels in each cancer (details not shown). A median of 31 indels (range 6–54) per tumour were potentially functional within coding regions (frameshift, stop-gain, stop-loss or splice site). We searched for regional SNV and indel hotspots (including ‘kataegis’) genome-wide within 1 Mb windows ( Supplementary Fig. 2 ). Most of the hotspot regions identified lay near centromeres and telomeres, probably reflecting the increased difficulty in mapping and calling variants there, but possibly resulting from impaired access of DNA repair machinery to these heterochromatic sites. We also identified several euchromatic mutation hotspots, but these could all be accounted for by (i) large duplicated regions prone to variant miscalling (generally present in many tumours) or (ii) local copy number increases (generally present in single cancers). We validated a subset of mutations using an Ion Torrent 150 cancer-gene panel (see Methods). Ninety-seven per cent of variants reported using the Illumina-Stampy–Playtpus pipeline were confirmed by the Ion Torrent technology. Structural variation All 14 cancers with genome-wide sequence data were analysed for copy number changes using OncoSNP-Seq. In addition, a sub-set of 10 cancers was analysed using Illumina Omni1M SNP arrays, with high concordance between the methods (median 75.6%). Somatic copy number changes were present in all 14 genomes ( Supplementary Fig. 3 ; Supplementary Data 1 ). The proportion of the genome showing copy number changes ranged from 12% (#4101) to 69% (#3034). Frequent large-scale copy number changes (found in six or more tumours) included gains of 1q, 3q and 8q, as well as loss of chromosome 9. Very few regions of high-level copy number gain were found, an exception being amplification around the CCND1 oncogene on chr11q13.3 and at the FGFR3 locus on chr4p16.3, each in a single cancer (#4121 and #615, respectively). Two cancers (#615 and #3008) had acquired homozygous deletions at the CDKN2A locus (chr9p21.3), and other homozygous deletions present in single cancers involved genes such as PPARGC1A, RFX3 and FAT1 ( Supplementary Table 2 ). With the exception of CDKN2A and FAT1 (see below), we found no good evidence from our own or The Cancer Genome Atlas (TCGA) mutation data to support the notion that any of the homozygously deleted genes acted as bladder cancer tumour suppressors. We specifically searched for chromosome arms that had undergone chromothripsis, which we defined for convenience as evidence of at least 10 copy number and/or loss of heterozyosity (LOH) transitions on a single arm. Cancer #745, which had the most chromosomally unstable genome of the tumours analysed, showed chromothripsis involving chromosome arms 3p, 5q, 6p and X ( Supplementary Fig. 4 ). Three other cancers had one or two arms with chromothripsis, but no recurrent region was observed across the set of 14 tumours. Using BreakDancer followed by specific quality filtering (see Methods), we found between 618 and 3,550 predicted inter-chromosomal breakpoints in each tumour. To reduce complexity, we focussed on anchor points lying within gene boundaries, resulting in a range of 18–86 inter-chromosomal changes per cancer ( Supplementary Data 2 ), although no anchor points lay within an exon. Driver genes For discovery of new bladder cancer-driver mutations, we restricted our analysis to protein-coding regions. In addition to our discovery set cancers, exome sequence data from one additional stage pTa bladder cancer were available, making a total of 15 bladder cancers analysed for driver gene detection. We filtered somatic mutations to exclude all base substitutions with moderate or benign predicted functional effects (Sorting Intolerant From Tolerant (SIFT) score >0.2 and Polyphen2 score <0.8). All protein-truncating and splice-site mutations were retained. We then removed from this list genes that were mutated in only one cancer. We inspected all mutant sequencing reads manually and excluded any of evidently poor local quality. 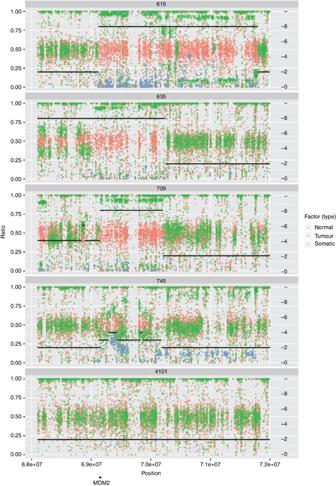Figure 3: TheMDM2amplicon. SNV allele frequencies (left-hand y axis) across each of the amplicons in the four cancers (#615, #635, #709 and #745) with copy number gain aroundMDM2are shown. The red dots correspond to variants present in the constitutional DNA, green to the same variants in the tumours and blue to somatic SNVs. Estimated copy number in each region (right-hand y axis) is shown as a black line for guidance, although close inspection of the allelic frequency changes suggests that the level of amplicon complexity is not fully captured. A tumour withoutMDM2region amplification (#4101) is shown for comparison. The position ofMDM2(chr12:69,201,971–69,239,320) is shown below the plots. Nineteen genes survived this process ( Table 3 ; Fig. 2 ), including several—for example, TP53 , FGFR3 , ARID1A and KDM6A —which at the time of analysis had previously been identified as bladder cancer-related genes [4] , [5] , [8] , [9] . Table 3 Known bladder cancer-driver mutations and other mutations in genes fulfilling the filtering criteria for further analysis. Full size table Figure 2: Summary of known and putative somatic-driver mutations after filtering in each cancer. MDM2 amplification is included in the figure for comparison with TP53 and CDKN1A. The established driver mutations PIK3CA and MLL3 are included despite being present in only one tumour to allow comparison with the presence of other mutations. Note that only mutations passing our filtering criteria are shown here, and that other potentially pathogenic mutations of lesser predicted functional effects may exist in these cancers. Full size image Prioritized genes that had not previously been reported as bladder cancer drivers included STAG2, B3GNT9, FAT1 and CDKN1A. We chose STAG2, MLL2/KMT2D and CDKN1A for further replication testing, based on the presence of at least one protein-truncating mutation and the paucity of mutations previously reported in cancers. Furthermore, all three genes were excellent functional candidates. STAG2 protein is required for the cohesion of sister chromatids after DNA replication and interacts directly with RAD21 in the cohesin complex. MLL2 is a histone methyltransferase. CDKN1A (p21 WAF1/CIP1 ) is a regulator of progression in G 1 and S phases of the cell cycle [10] , and is controlled by p53 in response to a variety of stress stimuli. p21 expression changes have been found in multiple tumour types, but mutations have very rarely been reported. We validated the STAG2 and CDKN1A changes detected by whole-genome sequencing using Sanger sequencing in the discovery set of tumours, and then undertook replication testing in a set of 35 additional bladder cancers ( Supplementary Table 3 ). 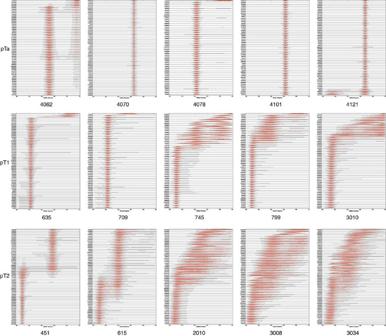Figure 4: Clonality across the tumours. Summary of the frequency distributions of the key somatic mutations plus 50 random SNVs (yaxis) for each tumour. Thexaxis shows the frequency of each mutant between 0 and 1. SeeSupplementary Data 3for more details. Four further protein-truncating and missense CDKN1A mutations were found ( Supplementary Table 4 ), and of the total of six CDKN1A- mutant cancers in our set, two (33%) showed LOH. One of the 35 replication cancers had a somatic mutation in STAG2. This was a splice-site change that we showed to affect mRNA splicing ( Supplementary Fig. 5 ). Subsequent to us performing this work, STAG2- and MLL2/KMT2D -driver mutations were reported in bladder cancers by other groups [4] , [5] , [6] , and we did not proceed to replication test MLL2/KMT2D in our own samples. Two of our 15 sequenced cancers had acquired nonsense mutations in FAT1 ( Table 3 ), which encodes a large protocadherin that contains multiple transmembrane repeats. One of these two cancers showed LOH at FAT1 . In addition, we detected a third cancer with predicted homozygous deletion of FAT1 ( Supplementary Table 2 ). Although testing of FAT1 was impractical in our replication samples owing to moderate DNA quantity and the large size of the FAT1 gene, we performed in silico replication using publicly available data from 99 bladder cancers in the TCGA consortium. That group’s data showed two tumours with protein-truncating FAT1 mutations and a further cancer with a missense change, p.Ile2276Met, predicted to have severe functional effects (SIFT=0.05, Polyphen2=0.87). We then examined all the bladder cancer-driver genes for mutations outside protein-coding regions. Two SNV mutations in untranslated regions were found, one in the 3′UTR of ARID1A and the other in the 3′UTR of FGFR3 , but neither had predicted effects on miRNA binding or mRNA structure (details not shown). No promoter mutations were detected. We then examined 50 kb regions around the driver genes for somatic mutations that might disrupt regulatory elements. On the basis of the reasoning that the most functionally profound changes were likely to involve severe disruption of regulatory regions or motifs, we focused on indels of ≥5 bp. A single change fulfilling these criteria was found, a 13-bp deletion upstream of FGFR3 (chr4:1,754,064; 5′-TCCCCCGCCCCAAC-3′>T) that removed a site shown to be methylated in multiple tissue types ( http://genome.ucsc.edu/ ). Pathway analysis ( Supplementary Fig. 6 ) reassuringly found ‘bladder cancer’ to be first in the list of mutated gene sets. Less expected were the findings that mutations in Wnt signalling, adherens junction and Notch signalling pathways were over-represented, given that none of the top driver mutations played principal roles in any of these processes. The MDM2 amplicon Our copy number assessment had identified a small, recurrent duplication/amplification on chromosome 12 (minimal region 69.1–70.0 Mb) that involved the MDM2 gene, a known driver oncogene in bladder cancer [11] and presumed target of the copy number gain ( Figs 2 and 3 ). None of our cancers, whether with or without copy number gain at this site, and no TCGA cancers harboured additional activating mutations in MDM2 . In addition to MDM2, genes contained within the amplicons included NUP107, CPM, CPSF6, LYZ, YEATS4 and FRS2. The chr12 duplication was present only in invasive lesions and, as expected, was mutually exclusive with TP53 mutations. The availability of whole-genome sequence allowed us to investigate the amplicon structure in detail, using copy number predictions and allele frequency data for both germline polymorphisms and somatic mutations ( Fig. 3 ). The amplicons in all four cancers had a proximal boundary close to chr12:69.1 Mb, although only two cancers appeared to share an identical breakpoint at this site. The distal amplicon boundary was more variable, ranging from chr12:70.2 to chr12:71.9 Mb ( Fig. 3 ). We noted that two regions of homology, to chromosomes 5q and 8q, lay close to the breakpoint sites, but we found no evidence of translocations between the MDM2 region and these sites. It appeared that all the amplicons resulted from local structural rearrangements. Figure 3: The MDM2 amplicon. SNV allele frequencies (left-hand y axis) across each of the amplicons in the four cancers (#615, #635, #709 and #745) with copy number gain around MDM2 are shown. The red dots correspond to variants present in the constitutional DNA, green to the same variants in the tumours and blue to somatic SNVs. Estimated copy number in each region (right-hand y axis) is shown as a black line for guidance, although close inspection of the allelic frequency changes suggests that the level of amplicon complexity is not fully captured. A tumour without MDM2 region amplification (#4101) is shown for comparison. The position of MDM2 (chr12:69,201,971–69,239,320) is shown below the plots. Full size image In none of the four cancers was the region of amplification structurally simple. Estimated copy number at MDM2 varied from 3 to 8. However, total copy number and allelic ratios varied along each amplicon, with intercalated regions of high- and low-level amplification. MDM2 was located in a region of high-level copy number (CN=8) in three of the four tumours (#615, #635 and #709), and within a region of single copy gain in the remaining tumour (#745). Allele-specific assessment within the amplicons ( Fig. 3 ) showed severe allelic asymmetry in the three cancers with high-level gain, suggesting that a single copy of chromosome 12 had become destabilized in the region. Somatic SNV and, particularly, indel frequencies were grossly elevated above background and had independently been identified as regions of possible kataegis ( Supplementary Fig. 2 ). The elevation in indel mutation numbers could not solely be accounted for by the increased total copy number, suggesting that it might be linked to the region’s instability in some way, although errors in mapping of chimaeric reads could not be excluded. The SNV mutation spectrum within the amplicon did not differ significantly from the genome-wide spectrum of each cancer ( Fig. 1 ). Overall, these data strongly suggested that a single copy of chromosome 12 had acquired a fundamentally destabilized region around MDM2 in at least three, and possibly four, tumours. TP53 and CDKN1A protein expression in bladder cancers Immunohistochemistry (IHC) was performed on 46 additional bladder cancer patients for both p53 and p21 proteins. Using cutoff points of 5, 10 or 20% of tumour cells displaying nuclear immunoreactivities for both proteins, we observed no significant correlation between TP53 and CDKN1A expression ( Supplementary Table 5 ; Supplementary Fig. 7 ). The results remained similar with full semi-quantitative scores. Evolution and clonal structure Clonal structure was evaluated using Pyclone, incorporating the bladder cancer-driver mutations and 50 random SNVs ( Fig. 4 ; Supplementary Data 3 ). Two pTa tumours (#4070 and #4101) showed only a single clonal cluster and three cancers (#4078, #709 and #4121) appeared monoclonal apart from one outlier. The other cancers showed good evidence of multiple clones, with a maximum number of 36 clonal clusters in tumour 3008. Tumour 451 was notable for its predicted early divergence into two clones, each distinct from the other but with high levels of similarity within each sub-clone. We tested the hypothesis that cancers with greater genetic diversity (larger numbers of sub-clones) would also have higher SNV/indel burden and/or a greater proportion of the genome showing copy number aberrations, and found that both were the case (Spearman’s ρ =0.83, P =0.0002 and ρ =0.61, P =0.021, respectively). Figure 4: Clonality across the tumours. Summary of the frequency distributions of the key somatic mutations plus 50 random SNVs ( y axis) for each tumour. The x axis shows the frequency of each mutant between 0 and 1. See Supplementary Data 3 for more details. Full size image Clinicopathological-molecular associations The number of cancers analysed by whole-genome sequencing was too low to reliably analyse associations between clinicopathological variables and specific mutations, although we noted that FGFR3 mutations were more common in pTa tumours, as expected. All invasive (pT1 and pT2) lesions had TP53, CDKN1A or CDKN2A mutations or MDM2 amplification, and none of these genes had changes in pTa tumours. We also tested for differences in mutation burden among the non-invasive, early invasive and muscle-invasive tumour groups. Since no measure of clonal structure or mutation burden differed significantly between pT1 and pT2 cancers ( P >0.15, N =10, Wilcoxon test), we combined these groups for further analysis. We found that the number of somatic mutations, the proportion of the genome affected by copy number changes (a surrogate for chromosomal instability) and the number of predicted sub-clones were all significantly positively associated with increasing stage ( P =0.0047, P =0.0046 and P =0.060, respectively; Wilcoxon test, pTa versus pT1/pT2). Grade (G1,2 versus G3), which was positively correlated with stage, was similarly associated with the same three molecular burden variables ( P =0.0041, P =0.0062 and P =0.0082). Age, sex and smoking status (ever versus never) were not associated with any of the three measures of mutation burden and diversity. Mutation spectra (proportions of different types of SNVs) were not in general associated with clinicopathological variables, including age and smoking history. One possible exception was the proportion of T:A>G>C changes, which was positively associated with higher stage ( P =0.037, Kruskal–Wallis test). Our whole-genome sequencing of bladder carcinomas of various sub-types has confirmed the known bladder cancer-driver genes, including our independent discovery of STAG2- driver mutations that have recently been reported by other groups [4] , [5] , [6] ( Table 3 ; Fig. 2 ). We additionally identified and replicated mutations in CDKN1A that are strongly predicted to impair protein function, in both our discovery and replication data sets. In some cases, these CDKN1A changes were accompanied by loss of heterozygosity. Our findings were further supported by inspection of TCGA exome sequencing data from 99 bladder cancers, which at the time of analysis in October 2013 showed two somatic SNVs in CDKN1A, one predicted to have strongly deleterious effects (p.Gly61Val, SIFT 0.00, Polyphen2 0.997) and the other to have possibly damaging effects (p.Asp136His, SIFT=0.11, Polphen2=0.553). Some years ago, Lacombe et al. [12] reported a single bladder cancer, out of 27 analysed, with a protein-truncating CDKN1A mutation, and we additionally note that contemporaneous TCGA bladder cancer exome sequencing data (January 2014) show 18 CDKN1A- mutant bladder cancers of a total of 130 analysed [13] . We conclude that CDKN1A is a tumour suppressor gene in bladder carcinoma, and we note that its inactivation is a bladder-specific change, since >1% of cancers of other sites harbour CDKN1A mutations ( http://cancer.sanger.ac.uk/cosmic/gene/overview?ln=Cdkn1a ). CDKN1A and CDKN2A mutations were mutually exclusive in both our and TCGA data. Although p21, the protein encoded by CDKN1A, acts downstream of p53, we found one cancer (#1992) from our full set of 50 tumours to have both CDKN1A (p.Tyr77del) and TP53 (p.Arg213Pro) mutations (details not shown) and another (#745) to have CDKN1A mutation (p.Trp65Arg) and low-level MDM2 amplification ( Supplementary Table 4 ). Interestingly, p21 protein has variably been described as having oncogenic and anti-oncogenic effects in a number of cancer types [14] . The genetic data strongly suggest that loss of p21 function promotes the growth of bladder carcinomas. Our genetic data also strongly suggest that loss of p21 function may augment defects caused by inactivation of p53, but does not act as a simple substitute. Our IHC data support this contention. Cancers with low or absent p53 might have various underlying causes (including not only protein-destabilizing TP53 mutations, MDM2 amplification, chr9p21 deletions involving p14 ARF , but also a normal p53 pathway. However, stabilization of p53 protein is generally accompanied by pathogenic missense TP53 mutations, and these cancers would not generally be expected to activate p21 expression [15] . The finding by ourselves and others [16] that a proportion of bladder cancers expresses both p53 and p21 suggests that p21 can be activated by a p53-independent pathway in these tumours, providing a rationale for some of them acquiring both p21 and p53 mutation. In addition to identifying CDKN1A mutations, we have highlighted inactivating FAT1 mutations as possible bladder cancer drivers, on the basis of protein-truncating mutations and deletions in our own and TCGA data. FAT1 is a tumour suppressor in Drosophila and an excellent candidate for having a similar role in humans. It functions in cell adhesion and is expressed in the urinary tract. However, FAT1 is an extremely large gene, and hence it is not yet possible to assign driver or passenger status to the mutations we have found. We additionally identified recurrent mutations in RYR2, FMN1, B3GNT9 and PIEZO2 in our discovery set of cancers, but the importance of these genes for bladder carcinogenesis remains uncertain. The mutation spectra of our bladder cancers did not closely match any of the 22 specific signatures previously reported, although there were similarities to signature 1b (ref. 7 ). Specifically, we did not find evidence of a carcinogen signature or a preponderance of G:C>C:G mutations reported in some bladder cancers [17] . The differences between the two data sets might in part result from the smaller size of our cohort, or from differences in the types of tumour sequenced, but we suggest that the G:C>C:G mutation signature is not common in bladder cancer. The use of genome-wide deep sequencing allowed us to perform extensive work on structural variations, including copy number changes and translocations. Although no recurrent translocations with intragenic breakpoints were found, several focal regions of deletion and gain were detected. Specifically, we characterized the structure of the recurrent amplification around MDM2 , which was found in 4 of 10 invasive tumours. This analysis showed that in most of these tumours, there was heterogeneity in copy number across the amplicon. Although there was no evidence of activating MDM2 mutations, amplification in most cancers was greatly asymmetric with respect to constitutional polymorphisms, suggesting that one copy of chromosome 12 became locally destabilized, leading to the observed rearrangements and, perhaps, an elevated frequency of small indels. Breakdancer analysis did not indicate the translocation of the MDM2 amplicon to any other chromosome, although we cannot exclude its location on double-minute chromosomes. There were clear associations between tumour stage and molecular features. In general, invasive tumours had larger burdens of mutations of all types, including SNVs and copy number changes. The invasive tumours also showed greater clonal diversity. With the possible exception of T:A>G>C changes, there was no clear association between stage and SNV mutation spectrum, suggesting that invasion was not driven by mutagen exposure or specific defects in DNA repair (although defects causing chromosomal instability remained a possible cause of invasive behaviour). It will be of interest for larger future studies to assess associations between molecular phenotypes, such as mutation burden, and other measures of bladder cancer behaviour, including prognosis. Furthermore, it will be important to test the scenario that some early-stage bladder cancers harbour sub-clones with p53 or p21 inactivation, and/or greater diversity and/or mutation burden, thus allowing the identification of tumours with a high risk of progression to invasive disease and permitting more appropriate and intensive management. Sample description Ethics approval was obtained from South Yorkshire Research Ethics Committee (project 10/H1310/73), Oxfordshire Research Ethics Committee C (project 09/H0606/5), Leeds (East) Research Ethics Committee (project 04/Q1206/62) and NRES Committee London-Bromley (project 13/LO/0540). The discovery set of tumour cancers with whole-genome sequence data comprised 14 bladder cancers, paired with peripheral blood, that had been collected from unrelated individuals presenting to the Urology Department, Royal Hallamshire Hospital, Sheffield, between June 2008 and September 2011. Four cancers were of low-grade papillary morphology (pTaG1-2: #4062, #4070, #4101 and #4121), five were high grade invading the lamina propria (pT1G3: #635, #709, #745, #799 and #3010, with #635 and #3010 subsequently becoming muscle invasive) and five were muscle invasive (pT2-pT3: #451, #615, #2010, #3008 and #3034). Exome sequence data were available from a further low-grade cancer, #4078. All tumours were sampled at transurethral resection or cystectomy and had not previously received any other therapy. The presence of at least 70% cancer cells in the tumour specimens was confirmed by routine histological assessment. Genomic DNA was extracted from each tumour and paired blood sample using standard methods. The replication set comprised 35 frozen biopsies of bladder carcinomas (16 pTa or pTis, 10 pT1G3, 9 pT2) from patients who had donated samples to the Oxford Radcliffe Biobank. Each sample was microdissected to maximize the amount of tumour, using haematoxylin and eosin-stained slides as a guide. After confirming that each specimen included a majority of cancer cells, DNA was extracted using standard methods of digestion with Laird’s lysis buffer plus proteinase K, followed by phenol–chloroform extraction and ethanol precipitation. For selected cancers where mutations were detected, the somatic origin of those changes was confirmed by microscope-guided dissection of normal tissue from the tumour specimen. The IHC set comprised samples from 46 patients with muscle-invasive bladder cancer, treated with radical radiotherapy at Leeds Teaching Hospitals NHS Trust from January 2006 to February 2009 as described in and one further patient. The median patient age was 76.5 years (range 57.8–86.5); 33 were male (72%) and 13 female (28%). Suitable invasive tumour areas were identified by a consultant histopathologist (SB) on haematoxylin and eosin sections from formalin-fixed paraffin-embedded bladder chips obtained at pre-radiotherapy transurethral resection. Up to five 0.6 mm tissue microarray (TMA) cores per patient were embedded into a single recipient block, from which 0.4 μM sections were taken for IHC staining. Whole-genome sequencing Sequencing in the discovery set was performed as part of the WGS500 project using a dedicated pipeline. Samples were quantified using the Qubit system (Invitrogen) and sequencing libraries constructed from 1 μg DNA using the NEBNext DNA Sample Prep Master Mix Set 1 Kit. Ligation of adaptors was performed using 6 μl of the Illumina Multiplexing Sample Preparation Oliogonucleotide Kit. Libraries were size selected using 2% gel electrophoresis and the distribution of fragments in the purified fraction was determined using the Tapestation 1DK system (Agilent/Lab901). Each library was PCR enriched using the following custom primers: Multiplex PCR primer 1.0: 5′-AATGATACGGCGACCACCGAGATCTACACTCTTTCCCTACACGACGCTCTTCCGATCT-3′; index primer: 5′-CAAGCAGAAGACGGCATACGAGAT[INDEX]CAGTGACTGGAGTTCAGACGTGTGCTCTTCCGATCT-3′. Indexes were 8 bp long and part of an indexing system developed in-house. Four independent PCR reactions per sample were prepared using 25% volume of the pre-PCR library each. After eight cycles of PCR (cycling conditions as per Illumina recommendations), the four reactions were pooled and purified with AmpureXp beads. The final size distribution was determined using the Tapestation 1DK system (Agilent/Lab901). The concentration of each library was determined by the Agilent qPCR Library Quantification kit. Samples were sequenced using the Illumina HiSeq2000 platform as paired 100 bp reads with Chemistry version 3.0, with the aim of a target average coverage of 30 × for the blood DNA and 60 × for the tumours. After removal of PCR duplicates using Picard, reads were mapped with Stampy version 1.0.12 (r975) [18] onto the Human Reference Genome (GRCh37d5/hg19). SNVs and small insertion–deletions (indels) were called with Platypus version 0.1.8 (ref. 19 ) using the tumour-normal pairs of bam files together to ensure comparable calls at every locus. Variants were only called if they were assigned a sufficiently high posterior probability (Phred score of 5). Additional filters were used to remove variants in low-quality reads. Although we removed the allele bias to increase sensitivity, we add filters on the number of high-quality reads at a location, carrying the variants and overall. Similarly, we made use of the difference between log likelihood ratios of each potential genotype to increase certainty. Finally, we made sure that the automatic call matched the data by expert visual inspection of the mapped reads onto the reference genome using read direction colouring on top of the standard Integrative Genomics Viewer (IGV) scheme ( http://www.broadinstitute.org/igv/alignmentdata/ ). Variants were annotated with ANNOVAR (RefSeq gene models) using: single nucleotide polymorphism database (dbSNP) (132); 1,000 genomes project allele frequencies (November 2011); University of California Santa Cruz (UCSC) segmental duplication scores; and UCSC 46 species conservation scores. Candidate variants were annotated with predictions of functional importance from SIFT and PolyPhen2. Owing to the possibility of copy number changes and intra-tumour genetic heterogeneity, we did not apply the default strand and allele bias filters to the data. However, we selected only variants at sites with at least 10 reads. First calls were compared between matched constitutional and tumour samples to identify somatic mutations. Known variants present at frequency >0.05 in the 1,000 Genome project, dbSNP or in the Exome Sequencing Project were also removed. Variants identified in constitutional DNA from any of the other non-cancer sequencing projects of the WGS500 consortium (29 million variants across 284 samples) were discarded as being more likely due to systematic error in our pipeline than genuine somatic mutation. Ion Torrent sequencing A custom 150 cancer-gene exome panel (details available on request) was used for technical validation of the whole-genome sequencing in the 15 bladder carcinomas. Approximately 100 ng DNA was used for sequencing. Mean read depth was 1,380. Variants present in the genome and exome sequence data were assessed alongside the equivalent Ion Torrent data, using both automatic calls in the Torrent Server output and visual inspection using the IGV. Targeted sequencing Validation and replication were performed with bidirectional Sanger sequencing of the coding regions of CDKN1A and of prioritized regions (exons 8–11 and 17–25) of STAG2 ( Supplementary Table 6 ). In addition, well-established methods were used to screen for mutations in exons 5–8 of TP53. Since neither CDKN1A nor STAG2 was present on the Ion Torrent cancer-gene exome panel, we also sequenced these genes in the 15 cancers with genome or exome sequence data. The somatic origin of any variation from the human reference sequence was confirmed by analysis of paired DNA from blood or normal urothelium. All PCR reaction conditions are available on request. Mutations were analysed with Mutation Surveyor V3.97 and confirmed by inspection of electropherograms. Splice-site mutation analysis To assess effects on mRNA splicing of the STAG2 mutation identified in the replication set of cancers, frozen bladder cancer was homogenized using the gentleMACS homogenizer (Miltenyi Biotec) and RNA isolated using TRIzol (Life Technologies). Bladder or pooled RNA from the First Choice Human RNA panel (Ambion) was used as a negative control. The RNA was treated with DNase I (Fermentas) to eliminate contaminating genomic DNA, and cDNA synthesis was performed using the iScript cDNA synthesis kit (Bio-Rad). Subsequently, PCR was performed on tumour or control cDNA using Phusion High Fidelity PCR master-mix (Thermo Scientific) and the products examined by minigel electrophoresis ( Supplementary Table 6 ). Structural variants For analysis of copy number, LOH and ploidy, we used the OncoSNP-Seq [7] program, which identifies variation based on read depth and allelic fraction under various models of stromal contamination and ploidy. After careful assessment of the data, we systematically chose the model with average ploidy of the non-neoplastic part of the tumour closest to 2. Results were compiled across the samples using the online version of GREVE to highlight recurrence of changes [20] . Breakdancer version 1.1.2 with default parameters was used to identify potential rearrangements, focusing on inter-chromosomal translocations. Results were first filtered for a score of 99, a minimum of 10 total supporting read pairs covering the breakpoints. Looking for functional rearrangement, we then reduced the list to breakpoints within genes and exons ( Supplementary Data 2 ). Single nucleotide polymorphism arrays Ten tumour:normal pairs (451, 615, 635, 709, 745, 799, 2010, 3008, 3010 and 3034) were genotyped using the Illumina Omni1 SNP array. The data were analysed using Genome Studio and OncoSNP [21] , and used to test the validity of the next-generation sequencing calls as well as the evaluation of copy number variation. Prediction of effects of exonic mutations outside coding regions MicroRNA binding was assessed by the TargetScan 6.2 program for mammals ( http://www.targetscan.org/ ) across conserved and partly conserved miRNA families. In addition, we examined the sno/miRNA track from the Human Genome Browser ( http://genome.ucsc.edu ) based on miRBase Release 15.0 (April 2010) and snoRNABase Version 3. mRNA structure was assessed using RNAfold (http http://rna.tbi.univie.ac.at/ ), using the default ‘minimum free energy and partition function option. In both cases, mutant and reference sequences were compared. Clonal structure Allelic heterogeneity, and thus clonal structure, was evaluated using PyClone version 0.12.3.1 (ref. 22 ). Allelic frequencies of selected somatic mutations were obtained using the number of reads and the number of reads carrying a variant as the total copy number. The copy number value at each of these loci and the tumour content were obtained from OncoSNP-Seq model selection as described above. We performed the clonal structure assessment using the three most likely values of each cancer’s DNA index from OncoSNP-Seq—the result from the estimate with the greatest likelihood is presented herein. Other DNA index estimates produced modest quantitative differences in clonal structure (data not shown), but these were insufficient to alter qualitative conclusions regarding clonality or to affect the analysis of clonal structure and clinicopathological features of the cancers. For each sample, a specific set of genome-wide somatic mutation was selected to characterize its heterogeneity: 50 randomly selected somatic mutations across the genome were added to the candidate somatic mutations. Pathway analysis Pathway analysis was performed using the online version of Intogen [23] using the annotated, quality filtered, somatic mutations from all 15 samples with genome-wide and exome-wide sequence data. Immunohistochemistry IHC analysis of p21 and p53 was carried out using a standard avidin–biotin–peroxidase technique. Briefly, TMA sections were dewaxed and rehydrated through xylene, graded ethanol and water. Endogenous peroxidase activity was blocked in 3% hydrogen peroxide for 20 min before heat-induced epitope retrieval at 110 °C for 1 min, in citrate buffer (10 mM citric acid, 0.05% Tween 20, pH 6.0) for p21 or Tris–EDTA buffer (10 mM Tris base, 1 mM EDTA solution, 0.05% Tween 20, pH 9.0) for p53 sections, and samples allowed to cool at room temperature to enhance antigen retrieval. After washing with running water and TBS, endogenous protein-binding activity was quelled using avidin–biotin blocking agent (Vector, Peterborough, UK) and 10% normal goat serum (Dako, Cambridgeshire, UK). Sections were incubated with primary antibody diluted in 1% BSA (VWR International, Leicestershire, UK) at optimized dilutions: anti-p21 (1:20, 12D1, Cell Signalling), anti-p53 (1:50,000, DO-1, Santa-Cruz), at 4 °C overnight. The Dako REAL Detection System Peroxidase/DAB+ Rabbit/Mouse kit was then employed to determine immunoreactivity, as per manufacturer’s instructions, with 1:50 (p21) and 1:200 (p53) dilutions of Dako REAL DAB+ Chromogen to Dako REAL HRP Substrate Buffer. Sections were washed, and then counterstained for 15 s in filtered Harris Haematoxylin (VWR, Leicestershire, UK), before further washing, dehydration and mounting in dibutylphthalate xylene (Leica, Peterborough, UK). Slides were scanned using the Aperio ScanScope CS2 digital slide scanner at × 40 magnification and viewed using Aperio Image Scope viewing software. Analysis of nuclear staining was made by two independent scorers by measuring the percentage of positively stained tumour cells. A consensus was reached for intensity by taking the mean if scores were within 20% of each other; otherwise, images were reviewed and a consensus reached. TCGA data TCGA somatic exomic mutation data from 99 ‘bladder urothelial carcinoma’ samples were obtained from the TCGA data portal ( https://tcga-data.nci.nih.gov/tcga/ ) on 31st October 2013. Accession codes: Whole genome sequence data for 14 bladder cancers have been deposited at the European Genome-phenome Archive (EGA, http://www.ebi.ac.uk/ega/ ), which is hosted by the EBI, under the accession code EGAS00001000738. How to cite this article: Cazier, J.-B. et al. Whole-genome sequencing of bladder cancers reveals somatic CDKN1A mutations and clinicopathological associations with mutation burden. Nat. Commun. 5:3756 doi:10.1038/ncomms4756 (2014).